Diverse uncultivated ultra-small bacterial cells in groundwater Bacteria from phyla lacking cultivated representatives are widespread in natural systems and some have very small genomes. Here we test the hypothesis that these cells are small and thus might be enriched by filtration for coupled genomic and ultrastructural characterization. Metagenomic analysis of groundwater that passed through a ~0.2-μm filter reveals a wide diversity of bacteria from the WWE3, OP11 and OD1 candidate phyla. Cryogenic transmission electron microscopy demonstrates that, despite morphological variation, cells consistently have small cell size (0.009±0.002 μm 3 ). Ultrastructural features potentially related to cell and genome size minimization include tightly packed spirals inferred to be DNA, few densely packed ribosomes and a variety of pili-like structures that might enable inter-organism interactions that compensate for biosynthetic capacities inferred to be missing from genomic data. The results suggest that extremely small cell size is associated with these relatively common, yet little known organisms. The 1996 report of a meteorite from Mars containing putative microbial cells that were widely considered to be too small to be organisms spurred a long debate about the existence of nanobacteria [1] . Over the following years, various publications proposed the existence of ‘nannobacteria’ (or nanobes) in terrestrial samples [2] , sometimes with implied medical [3] and environmental [2] significance. However, a lack of solid biological evidence for the existence of cells considered to be too small to accommodate sufficient genomic DNA, RNA, proteins and solvent for life consigned nanobacteria to the scientific fringe (‘the cold fusion of microbiology’ [4] ). Other studies have documented the existence of ultramicrobacteria [5] , [6] or dwarf cells [7] , [8] , which may be in a starved, inactive state [9] . Some estimates suggest a minimum viable cell diameter of 0.25–0.30 μm including the bounding membrane and wall [10] (0.008–0.014 μm 3 volume) is required for life; another report suggested a minimum cell volume in the range of 0.014–0.06 μm 3 (ref. 6 ). Very recently, ultra-small bacteria with cell volumes of 0.013 μm 3 estimated from flow cytometry–fluorescence in situ hybridization (FISH) techniques were reported for marine Actinobacteria [11] . However, data are lacking for direct electron microscopic evidence for bacteria within and smaller than these size ranges. Interestingly, there is electron microscopic information for one lineage of nanoarchaea with average cell volumes in the range of 0.009–0.04 μm 3 (ref. 12 ). Recent evidence hints at the existence of bacteria in this same size range. Separate studies applied 16S ribosomal RNA (rRNA) gene [13] and metagenomic sequencing [14] to groundwater filtrates to demonstrate enrichment for some members of ‘candidate phyla’ (CP), branches of the bacterial domain lacking isolated representatives [15] . Notably, the complete and near-complete genomes of several CP bacteria recovered from filtrates of acetate-amended groundwater [14] and in the sediment [16] from an aquifer at Rifle, Colorado, USA were comparatively small, a feature expected if cells are small. Intriguingly, the genomes lack many biosynthetic capacities, suggesting a dependence on other microbial community members for many metabolic resources [16] . Here, we repeated the acetate amendment experiment of ref. 14 and recovered cells that passed through a ~0.2-μm filter for DNA extraction and phylogenetic characterization. We preserved cells in vitreous ice on site for later ultrastructural characterization using cryogenic transmission electron microscopy (cryo-TEM) [17] . Filtration enriched for cells of the WWE3, OP11 and OD1 phyla, a vast phylogenetic radiation that lacks cultivated representatives. We report cell characteristics, including the average cell size, and describe ultrastructural features that may be related to cell size minimization. Data collection and procedures Cells were recovered from groundwater prior to, and following acetate amendment for coupled metagenomic and ultrastructural characterization. In this study, we focused primarily on a sample of acetate-amended groundwater. However, we also obtained metagenomic information for a sample of groundwater collected from the same site prior to acetate injection to evaluate the impact of the acetate treatment on community composition. Cells that passed through a ~1.2-μm filter were collected on a ~0.2-μm filter and those that passed through the ~0.2-μm filter were collected on a ~0.1-μm filter. DNA was extracted from both filters for phylogenetic analysis. Cells that passed through the 0.2-μm filter from samples taken 7 and 9 days after acetate injection began were preserved in vitreous ice on site for later ultrastructural characterization using cryo-TEM [17] . Cryogenic preservation eliminates fixation and dehydration artefacts [18] and can provide morphological information with ~2–4 nm resolution [19] . To correlate molecular and cryo-TEM data, the same groundwater sample (GWB1, post-0.2 μm filtrate, collected 7 days after acetate injection) was analysed by cryo-TEM and metagenomics. Most bacteria belong to the WWE3, OP11 and OD1 phyla Analysis of 16S rRNA gene sequences from a clone library and reconstructed from metagenomic reads via EMIRGE [20] indicated that both size fractions were dominated by bacteria ( Fig. 1a,b ). We also profiled the overall community composition of the acetate-amended sample (GWB1) using all assembled sequences >5 kb in length and confirmed that the majority of sequences were from bacteria ( Supplementary Fig. 1 ). The composition of the community on the ~0.1-μm filter was markedly different to that collected on the ~0.2-μm filter ( Fig. 1a ; Supplementary Fig. 2 ). The majority of the bacteria on the ~0.1-μm filter were members of the WWE3, OP11 and OD1 CP ( Fig. 1a ; Supplementary Fig. 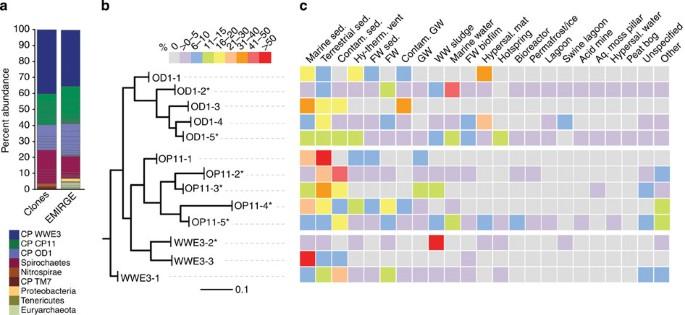Figure 1: Characterization of WWE3-OP11-OD1 radiation phylogeny and ecology. (a) Phylum level breakdown of the 16S OTUs recovered from 0.1-μm filter DNA Clone Library and EMIRGE reconstructions. CP, candidate phyla. (b) The tree contains the WWE3-OP11-OD1 16S rRNA gene sequences from the Arb-Silva database and our EMIRGE/Clone Library 0.1-μm filter sequences (n=1,523 sequences from the Arb-Silva database plus 49 sequences from the Rifle site). The tree is collapsed into ‘class’-level monophyletic groups; asterisks denote monophyletic groups to which Rifle sequences belong. (c) The coloured tiles represent environments from which sequences in each class were recovered, with colours corresponding to the percentage of each class found in the given environment. Sed., sediment; Contam., contaminated; Hy-therm., hydrothermal; FW, freshwater; GW, groundwater; WW, wastewater; Hypersal., hypersaline; Aq., aquatic. 3 ; Supplementary Table 1 ). Organisms from these lineages have been reported previously from a wide diversity of environment types ( Fig. 1c ). Figure 1: Characterization of WWE3-OP11-OD1 radiation phylogeny and ecology. ( a ) Phylum level breakdown of the 16S OTUs recovered from 0.1-μm filter DNA Clone Library and EMIRGE reconstructions. CP, candidate phyla. ( b ) The tree contains the WWE3-OP11-OD1 16S rRNA gene sequences from the Arb-Silva database and our EMIRGE/Clone Library 0.1-μm filter sequences ( n =1,523 sequences from the Arb-Silva database plus 49 sequences from the Rifle site). The tree is collapsed into ‘class’-level monophyletic groups; asterisks denote monophyletic groups to which Rifle sequences belong. ( c ) The coloured tiles represent environments from which sequences in each class were recovered, with colours corresponding to the percentage of each class found in the given environment. Sed., sediment; Contam., contaminated; Hy-therm., hydrothermal; FW, freshwater; GW, groundwater; WW, wastewater; Hypersal., hypersaline; Aq., aquatic. Full size image Genomic data indicated that Archaea comprise only a small fraction of the community, even when composition is profiled out to low abundance levels ( Supplementary Table 1 ). 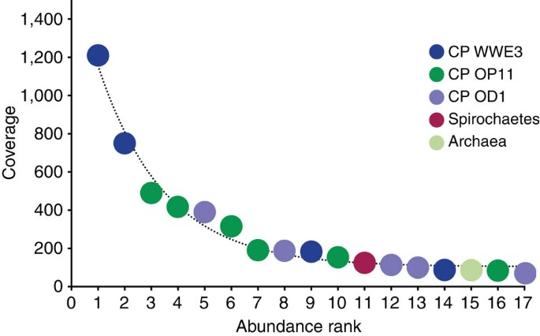Figure 2: Rank abundance curve illustrating dominance of the GWB1 microbial community (after acetate amendment) by WWE3 bacteria, with lower abundances of OP11, OD1 bacteria, Spirochaetes and archaea. Sequence coverage (yaxis) is directly related to organism abundance. Coverage values were computed by read mapping to contigs generated in two subassemblies. In some cases, coverage values were only available from one subassembly. We also used synchrotron-based infrared spectromicroscopy to estimate the fraction of cells that were bacteria versus archaea ( Supplementary Table 2 ; Supplementary Fig. 4 ; Supplementary Note 1 ). Bacterial membrane lipids consist of fatty acids with long alkylic (−CH 2 −) chains that have only one to two terminal methyl (−CH 3 ) groups, whereas archaeal membrane lipids consist of branched and saturated hydrocarbon isoprene, and therefore relatively less −CH 2 − and more −CH 3 groups [21] . We calculated the ratio of the infrared absorbance in the CH 3 region (2,990–2,945 cm −1 ) to that of the CH 2 region (2,945–2,900 cm −1 ) for cells from the same set of grids used for TEM analysis. Following criteria previously established [22] , we found that 97.2% (±4.4%) of the spectra derived from bacteria, whereas 2.8% of the spectra (±4.4%) were non-bacterial. We compared the metagenomic information for sample GWB1 with that of the microbial community composition in filtered groundwater prior to acetate injection (GWA1). Interestingly, the same CP bacterial groups are highly represented in both samples ( Fig. 2 ; Supplementary Figs 1 and 5 ; Supplementary Tables 3–5 ). Figure 2: Rank abundance curve illustrating dominance of the GWB1 microbial community (after acetate amendment) by WWE3 bacteria, with lower abundances of OP11, OD1 bacteria, Spirochaetes and archaea. Sequence coverage ( y axis) is directly related to organism abundance. Coverage values were computed by read mapping to contigs generated in two subassemblies. In some cases, coverage values were only available from one subassembly. Full size image Cell volumes close to the minimum expected size We surveyed hundreds of cells (for selection of targets for tomographic analysis) and recorded over 100 high-quality two-dimensional (2D) cryo-TEM images to profile the average cell diameter in the samples characterized by metagenomics ( Supplementary Note 2 ; Supplementary Table 6 ). The vast majority of cells were very small. Given the extensive cryo-TEM data set and deep metagenomic analysis (for example, Supplementary Fig. 1 ), it is statistically valid ( Supplementary Table 7 ) to conclude that the cells of the WWE3, OP11 and OD1 phyla that dominate the GWB1 filtrate are all extremely small. Morphotypes are illustrated in Supplementary Fig. 6 (see also Supplementary Fig. 7 and Supplementary Note 3 ). On the basis of 13 cryo-electron tomography three-dimensional (3D) reconstructions, the median of the cell’s longest dimension ( x axis) is 322.6±64.7 nm, intermediate dimension ( y axis) is 242.5±32.9 nm and shortest dimension ( z axis) is 189.7±22.0 nm ( Table 1 ). The median cell volume is 0.009±0.002 μm 3 including the cell wall and associated surface layer (S-layer) ( Fig. 3a ; Supplementary Fig. 8a ). The equivalent spherical diameter is 253±25 nm. The median cytoplasmic volume of the cells analysed by cryo-TEM is 0.005±0.002 μm 3 ( Table 2 ). Table 1 Size distribution of WWE3-OP11-OD1 ultra-small bacteria. 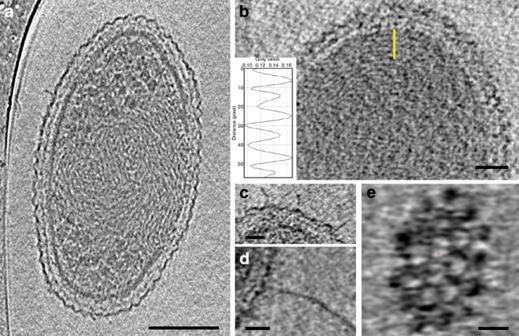Figure 3: Cryo-electron tomography images from 3D reconstructions of ultra-small bacteria. (a–e) One-voxel-thick slices. (a) 3D reconstruction reveals a very dense cytoplasmic compartment and a conspicuous, complex cell wall enveloped by a periodic surface layer (S-layer). The high contrast sub-cellular bodies located at cell ends are putative ribosomes. Scale bar, 100 nm. The full reconstruction is provided inSupplementary Movie 1. (b) Within the cytoplasm, periodic fringes (normal to yellow line) display a 5.6-nm spacing (see insert), consistent with tightly packed DNA. Scale bar, 50 nm. (c,d) Pili-like structures associated with cell surfaces. Scale bars, 20 nm. The full reconstruction fordis provided inSupplementary Movie 2. (e) Top view of the repeating unit of the S-layer. Scale bar, 20 nm. Full size table Figure 3: Cryo-electron tomography images from 3D reconstructions of ultra-small bacteria. ( a – e ) One-voxel-thick slices. ( a ) 3D reconstruction reveals a very dense cytoplasmic compartment and a conspicuous, complex cell wall enveloped by a periodic surface layer (S-layer). The high contrast sub-cellular bodies located at cell ends are putative ribosomes. Scale bar, 100 nm. The full reconstruction is provided in Supplementary Movie 1 . ( b ) Within the cytoplasm, periodic fringes (normal to yellow line) display a 5.6-nm spacing (see insert), consistent with tightly packed DNA. Scale bar, 50 nm. ( c , d ) Pili-like structures associated with cell surfaces. Scale bars, 20 nm. The full reconstruction for d is provided in Supplementary Movie 2 . ( e ) Top view of the repeating unit of the S-layer. Scale bar, 20 nm. Full size image Table 2 Cell volume and morphological features of WWE3-OP11-OD1 ultra-small bacteria. Full size table Ultrastructure and architecture of ultra-small bacteria Space optimization strategies are evident in the 3D architecture of the cells. Electron tomograms indicate relatively centrally located, large spiral structures ( Fig. 3a , best seen in Supplementary Movie 1 and Supplementary Fig. 8a ), some with a 5.6-nm periodicity ( Fig. 3b ). This periodicity, and the volume of these spiral structures ( Table 2 ), is consistent with tightly packed genomic DNA [23] . Several data sets suggest the presence of two interlinked coils, spiralling counter clockwise (see the first half of Supplementary Movie 1 ). Rounded objects of diameter ~20 nm ( Fig. 3a ; Supplementary Fig. 8b ; Supplementary Movie 1 ) are identified as ribosomes based on shape, contrast and size [24] . We observed that ribosomes are generally concentrated at cell ends; in some views, they appear to be regularly packed ( Supplementary Fig. 8b ). Such packing may indicate that ribosomes exist in tightly coordinated structures previously described as polysomes [25] . On average, cells contain 42±9.5 putative ribosomes ( Table 2 ). Most cells lack an outer membrane that would be expected for a Gram-negative cell envelope. Many have pili-like structures with a variety of lengths and thicknesses (for example, Fig. 3c ) that could confer motility ( Fig. 3d ; Supplementary Fig. 8a ; Supplementary Movie 1 ). Typically, the cell walls have an intriguing architecture, with a thick cytoplasmic membrane and a remarkable, distinct S-layer with a hexagonal symmetry ( Fig. 3e ; Supplementary Fig. 9 ; Supplementary Note 4 ) that appears to be anchored through the peptidoglycan to the cytoplasmic membrane ( Supplementary Figs 10 and 11 ; Supplementary Note 5 ). Given the small cell sizes, the large fractions of the cell volumes devoted to the cell walls, including the S-layers, suggest that these features are important for survival, possibly by mediating cell–cell interactions. Some S-layers are decorated with pili-like structures that are evenly distributed across the cell surface ( Fig. 4a ); in other cases the pili-like structures are sparsely distributed ( Supplementary Fig. 8a ). Slices from tomographic reconstructions indicate pili-like structures that pass through the cell wall into the cytoplasm ( Supplementary Fig. 12a ) and enigmatic ring-like structures associated with filaments within cells ( Supplementary Fig. 12b ). In some cases, long pili-like structures appear to link very small cells to larger cells ( Fig. 4b ; Supplementary Fig. 13 ). A cell surface-based interaction occurs between an ultra-small cell and a large cell that is inferred to be Spirochaete based on cell morphology (including an axial filament), metagenomic and clone library information ( Fig. 4c ; Supplementary Fig. 14 ). 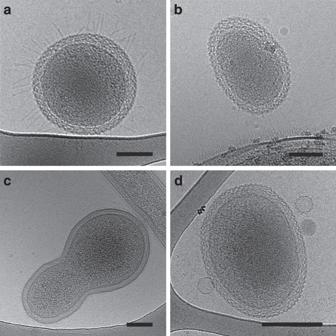Figure 4: Cryo-TEM images (2D) documenting morphology, size and some morphological features of ultra-small bacteria. The cell envelope includes a remarkable and distinct S-layer. Pili-like structures are clearly discernible: numerous radiating pili-like structures cover the surface of the cell ina, whereas polar pili-like structures occur on the cell inb, apparently connecting it to an adjacent bacterium (only part of the bacterium shown). (c) A dividing ultra-small bacterium in contact with a Spirocheate cell (only small region shown; also seeSupplementary Fig. 14). Note the contrast at the interface, suggesting cell-to-cell interaction. Three bacteriophages are associated with the surface of the cell ind. Scale bars, 100 nm. Figure 4: Cryo-TEM images (2D) documenting morphology, size and some morphological features of ultra-small bacteria. The cell envelope includes a remarkable and distinct S-layer. Pili-like structures are clearly discernible: numerous radiating pili-like structures cover the surface of the cell in a , whereas polar pili-like structures occur on the cell in b , apparently connecting it to an adjacent bacterium (only part of the bacterium shown). ( c ) A dividing ultra-small bacterium in contact with a Spirocheate cell (only small region shown; also see Supplementary Fig. 14 ). Note the contrast at the interface, suggesting cell-to-cell interaction. Three bacteriophages are associated with the surface of the cell in d . Scale bars, 100 nm. Full size image A decrease in cell size can occur if bacteria are exposed to low nutrient or starvation conditions (see reviews [5] , [6] ). Although nutrition status could impact cell size for the bacteria studied here, small size is predicted for normal cells, based on the sizes of complete WWE3, OP11 and OD1 bacterial genomes [16] . Notably, the cell in Fig. 4c has a dumbbell shape, suggesting that it is either dividing or budding. This is an indication that cells are active, not in a spore-like state. Further, some images indicate the presence of bacteriophage associated with cell surfaces ( Fig. 4d ), possibly also an indication that the cells are metabolically active. Thus, we conclude that small cell size is an inherent characteristic of these bacteria. We designed catalysed reporter deposition FISH (CARD-FISH) probes to specifically target rRNA sequences recovered via the clone library analysis ( Supplementary Table 8 ). As positive controls, the rRNA sequences were engineered onto plasmids carried by Escherichia coli cells [26] . Despite optimization of WWE3, OP11 or OD1 CARD-FISH probe hybridization conditions and successful labelling of the positive controls, regions with a fluorescence signal (that normally would be interpreted as labelled cells) could not be associated with cells when those same regions were visualized by cryo-electron microscopy. The failure to label cells is probably the consequence of the very low numbers of ribosomes per cell, but it might also be due to the tight ribosome packing, which could preclude probe access. Furthermore, the cell envelope may present a boundary that does not allow the penetration of the probes into the cells (see Supplementary Note 6 ). The cells could have been also lost during specimen transfer. More than half of the recognized bacterial phyla lack an isolated representative suitable for physiological and morphological characterization. Consequently, there are large gaps in our understanding of microbial biology. The first significant genomic sampling of multiple bacterial candidate phyla, including those studied here, suggested that these organisms have small genomes [14] . Very recently, Kantor et al. [16] confirmed this prediction reporting a complete genome for a WWE3 population that was 0.878 Mb in length, and a near-complete genome for a OD1 population of 0.694 Mb in length. A complete 0.984-Mb genome of an OD1 bacterium from the GWB1 sample and four complete OP11 genomes of ~0.820 to 1.050 Mb in length from the same experiment will be reported separately (C. Brown et al. , unpublished). Similarly, two recently reported complete genomes of TM7 CP bacteria were 0.845 and 1.013 Mb in length [16] , [27] . Here, we augment these findings by showing, via integrated clone library and metagenomic analyses, that WWE3, OP11 and OD1 cells can be enriched by filtration and that the cells are ultra-small ( Figs 1a and 2 ; Supplementary Fig. 2 ). There is generally a linear relationship between genome length (and number of protein-coding genes per genome) and cell size [28] . Notably, our cryo-TEM data show that the whole-cell sizes and also the cytoplasmic volumes ( Tables 1 and 2 ; Supplementary Table 6 ) are close to, and in some cases smaller than previous estimates for the lower size limit for life [6] , [10] . A bacterium that is growing and dividing needs to be large enough to accommodate DNA and RNA, enzymes for replication, transcription and translation, solvent, a minimum set of proteins and space to run these operations. A National Academy of Sciences workshop report addressed the question of the size limits for very small microorganisms [10] . In the calculations, the authors assumed a minimum of 250–450 proteins along with the genes and ribosome(s) necessary for their synthesis, and suggested a minimum cell size of 0.25–0.3 μm in diameter. One theoretical calculation assumed 100 non-ribosomal protein species and that each is present in only 10 copies, 1 ribosome, 1 transfer RNA set and 1 messenger RNA for each protein species and predicted a diameter (without a cell wall) of 186 nm (0.003 μm 3 ); another using 950 non-ribosomal proteins predicted a diameter (without a cell wall) of 339 nm (volume of 0.020 μm 3 ). Our data indicate that the CP cells studied here typically have 34–59 ribosomes. A single active ribosome, if surrounded by membrane and cell wall, occupies a sphere of 50–60 nm in diameter [10] . A space capable of holding 42 tightly packed ribosomes (diameter of 50 nm) would be close to 0.002 μm 3 in volume. Tightly packed genomic DNA (0.878 Mb for WWE3) should account for 0.001 μm 3 . On the basis of a median cytoplasmic cell volume of 0.005 μm 3 ( Table 2 ) measured in the current study, there would be ~0.002 μm 3 for other components and cell functioning. The WWE3, OP11 and OD1 genomes are smaller than genomes typical of free-living cells [14] , [16] . A large fraction of the genes encode hypothetical proteins, and apparently many pathways for core biosynthetic capacities expected in free-living cells were not detected [14] , [16] . Although the possibility of novel metabolic pathways cannot be ruled out, it was suggested that the organisms are at least partially dependent on another community member (or members) for basic metabolic building blocks [16] . For example, the organisms may be symbionts of other community members. Features expected in symbionts include small genome size, AT bias and loss of biosynthetic pathways [29] , [30] . Recently, McLean et al. [31] reported a similarly small genome for a member of the TM6 CP and suggested that the organism is a symbiont, and Gong et al. [32] showed that an OD1 bacterium occurs intracellularly in a protist. Interestingly, pili genes are well represented in the WWE3, OP11 and OD1 genomes [14] , [16] . For example, WWE3 and OD1 genomes encode components for type-IV pili, including pilT for twitching motility and several predicted pilins [16] . The pili genes are homologous to type-IV pili genes sometimes involved in the uptake of environmental DNA [33] , [34] and may aid the cells in inter-organism interactions and interacting with the environment [34] . TEM images recorded in the current study confirm the existence of these structures on cell surfaces, in some cases at high abundance levels. Interestingly, some long pili-like structures link very small cells to larger cells ( Fig. 4b ; Supplementary Fig. 13 ). This linkage is suggestive of a close association of some type. Pili-based associations described as nanowires have been suggested to play roles in electron transfer among different organisms (for example, ref. 35 ). Interestingly, physical association of different cell types via pili is distinct from the interaction mechanism reported previously for nanoarchaea with other cells inferred to be their hosts. For example, ARMAN nanoarchaea display a highly unusual association that involves direct penetration of the cell by a cytoplasmic extension from a nearby Thermoplasmatales cell [28] . In the case of Nanoarchaeum equitans , the nanoarchaea attach directly to the surface of their host Igniococcus cells in an obligate symbiotic relationship [36] . The abundance of glycosyl transferase genes in the OD1 and particularly the WWE3 genomes suggests the organisms devote significant energy to production of polysaccharides, glycoproteins and/or a glycosylated S-layer [16] . Furthermore, the OD1 genome contains a complete pathway for peptidoglycan synthesis [16] . Sortases, which covalently attach surface proteins to the cell wall of Gram-positive bacteria, and predicted sorted proteins are present in the WWE3 genome [16] . WWE3 and OD1 lack the outer membrane proteins typically found in type-IV secretion systems and do not make lipid A or lipopolysaccharide; thus the cell envelope is probably not similar to that of Gram-negative bacteria [16] . Consistent with metagenomic predictions, cryo-electron tomograms indicate that most cell types have cell envelopes with ultrastructural characteristics that are most similar to those of Gram-positive bacteria. The S-layer type cannot be clearly classified from the available data, but in Gram-positive bacteria and in certain archaea, the S-layer is non-covalently bound to cell wall components such as peptidoglycan, secondary cell wall polymers or pseudomurein. In most archaea, the S-layers exhibit pillar-like structures on the inner surface, which are involved in anchoring the arrays in the underlying cytoplasmic membrane [37] , [38] . Therefore, the cell envelope of the ultra-small bacteria studied here (thick cytoplasmic membrane, S-layer with a hexagonal symmetry and connectors) is inferred to have mixed character, sharing aspects of both Gram-positive bacteria and archaea cell envelopes. The three lineages now described as the WWE3, OP11 and OD1 phyla, originally part of a single CP [39] , [40] , are now recognized as part of a CP radiation that includes at least 14 possibly monophyletic phyla [41] . Members of this radiation have been detected in a wide variety of ecosystems ( Fig. 1c ). Given the wide evolutionary scope of this radiation, it is not surprising that we observed considerable morphological variation ( Fig. 1a,b ; Supplementary Figs 3 and 6 ; Supplementary Table 1 ). Extrapolating based on the information now on hand, this radiation may have maintained (over long evolutionary time) cells with consistently very small genomes, sparse metabolic capacities and very small cell sizes. The small cytoplasm space, tight packing of DNA into spirals, low number of ribosomes and reliance on other community members for basic metabolic requirements may be a broadly relevant strategy for size minimization. Slow growth rates (predicted based on low ribosome counts) and likely dependence on other organisms in the community, could well explain why members of these phyla have, to date, evaded cultivation. Field experiment and sample collection The research site near the town of Rifle, northwestern Colorado (USA), has been described previously [42] . Briefly, the site is located on a 9 ha floodplain in northwestern Colorado that is underlain by an aquifer comprised of 6–7 m of unconsolidated sands, silts, clays and gravels deposited by the Colorado River. Amendment of acetate to the aquifer occurred through five boreholes oriented orthogonal to groundwater flow direction and spaced at 1.5-m intervals. Cross-well mixing was used to disperse the injectate across the width of the injection zone. Groundwater samples were taken prior to (GWA1) and following acetate amendment (GWB1). Acetate-amended groundwater was injected upgradient 3.5 and 5.5 m below the surface to achieve aquifer concentrations of 15 mM (acetate; Sigma-Aldrich, Saint Louis, MO, USA) and 2 mM (bromide; Sigma-Aldrich). Prior to acetate amendment 140 l, and on 03 September 2011 and 05 September 2011, 7 days (GWB1) and 9 days after the start of acetate amendment, 100 l of groundwater were pumped and filtered sequentially through a 1.2-μm pore size pre-filter (293-mm diameter Supor-1200 hydrophilic polyethersulfone membrane disc filter; Pall Corporation, Ann Arbor, MI, USA), with biomass retained on a 0.2-μm pore size (293-mm diameter Supor-200 hydrophilic polyethersulfone membrane disc; Pall Corporation) and a 0.1-μm pore size sample filter (142-mm diameter Supor-100 hydrophilic polyethersulfone membrane disk filter; Pall Corporation). Filters were immediately frozen in an ethanol–dry ice mix, stored at −80 °C and shipped overnight to the University of California, Berkeley, for DNA extraction. For cryo-TEM, 500 ml of 0.2-μm filtrate was concentrated with Vivaspins (cutoff 30 kDa; GE Healthcare, Pittsburgh, PA, USA) to ~500 μl and cryo-plunged immediately (see below). For molecular, metagenomic and cryo-TEM correlation analyses, the same groundwater sample (GWB1) was used. DNA extractions Approximately 1 g of each filter was used for DNA extraction using the PowerMax Soil DNA Isolation kit (Mo Bio Laboratories Inc., Carlsbad, CA, USA, Cat# 12988). Manufacturer’s protocol was followed, with the exception of adding a freeze/thaw step and vortexing bead tubes for 3.5 min after addition of the SDS reagent, followed by 30 min at 65 °C with intermittent shaking. DNA in the 5-ml eluted volume was concentrated by sodium acetate/ethanol precipitation with glycogen followed by resuspension in provided elution buffer. Preparation of clone libraries and sequencing Full-length, bacterial 16S rRNA sequences were amplified by utilizing a gradient PCR using general bacterial primers 27F (5′-AGAGTTTGATCMTGGCTCAG-3′) and 1492 R (5′-GGTTACCTTGTTACGACTT-3′) [43] . For PCR, the thermocycler reaction conditions were as follows: initial denaturation at 94 °C for 1 min, 25 cycles of denaturation at 94 °C for 30 s, annealing across an eight-step gradient from 48–59 °C for 30 s, extension at 72 °C for 1 min and a final extension at 72 °C for 7 min. Correct amplicon size was verified with gel electrophoresis and the PCR product was cleaned up using the UltraClean PCR Clean-up Kit (Mo Bio Laboratories Inc., CA Cat# 12500). Clone libraries were generated using a TOPO TA cloning kit and electrocompetent cells (Life Technologies Corp., Grand Island, NY, USA). One hundred transformants from the 0.1- and 0.2-μm clone libraries were verified by colony PCR using the M13 forward (5′-GTAAAACGACGGCCAGT-3′) and reverse (5′-CAGGAAACAGCTATGAC-3′) primers and gel electrophoresis. The colony PCR thermocycler amplification conditions were as follows: E. coli cell lysis and initial denaturation at 95 °C for 10 min, 25 cycles of denaturation at 95 °C for 30 s, annealing at 53 °C for 30 s and extension at 72 °C for 1.5 min and a final extension at 72 °C for 7 min. Successful transformants were Sanger sequenced using the M13 forward and reverse primers (only for the 0.1-μm filter). Sequences were primer and vector screened using cross_match ( http://www.phrap.org ) and NCBI VecScreen ( http://www.ncbi.nlm.nih.gov/VecScreen/VecScreen.html ), quality scored using Phred ( http://www.phrap.org ) and assembled into contigs using Phrap ( http://www.phrap.org ). Sequences were trimmed to retain only bases Phred ≥q20 and high-quality contigs were tested for chimeras using USEARCH 64 ( http://www.drive5.com ). Sequences were identified utilizing BLAST [44] against the Arb-Silva Database ( http://www.arb-silva.de ). 16S rRNA gene phylogenetic analysis 16S rRNA gene sequences from cells retained on the 0.2 μm filter (50 clones, resulting in 21 operational taxonomic units (OTUs) after chimera checking and clustering as described previously) and 0.1-μm filter (108 clones, resulting in 24 OTUs) were obtained by sequencing of the clone libraries. The individual clone sequences were clustered at 97% using UCLUST (part of USEARCH 64). We also used EMIRGE [20] to reconstruct 16S rRNA gene sequences after trimming the Illumina reads using sickle to remove low-quality bases ( https://github.com/najoshi/sickle ). For EMIRGE, paired-end reads, where both reads were at least 60 nucleotides in length after trimming, were used as inputs. For each sample, EMIRGE was run for 100 iterations. Reconstructed sequences for all sampled taxa were combined with database sequences representing the most closely related taxa for subsequent analysis. EMIRGE reconstructions generated 26 and 36 OTUs for the 0.2- and 0.1-μm filters, respectively. EMIRGE, clone library and Arb-Silva database WWE3-OP11-OD1 16S rRNA gene sequences were aligned with MUSCLE [45] using default parameters. The alignment was used to generate a maximum likelihood tree with RAxML [46] using the GTRCAT model of nucleotide substitution and 200 bootstrapped replicates and E. coli as an outgroup. The tree was edited using iTOL [47] . Poorly aligned or lower-quality sequences from the Arb-Silva database were removed prior to further analysis. The environments from which each sequence was obtained were pulled from the Arb-Silva database using the Arb software package. Metagenomics methods A total of 9,781,022,700 bp of Illumina data (150 bp paired reads) was generated for GWA1 and 369,257,200 bp was generated for GWB1at the Joint Genome Institute, Walnut Creek, CA. The same GWB1 sample (0.1-μm filter fraction) was used for cryo-TEM characterization. Sequence data sets were assembled (after trimming to remove low-quality bases) using idba_ud [48] using the default settings. Open-reading frames were predicted using Meta-Prodigal [49] and assigned a preliminary annotation using USEARCH [44] against the Uniref90 database ( http://www.uniprot.org/ ). Community composition was profiled primarily using single-copy ribosomal protein S3 genes carried on scaffolds >5 kb in length (detection limit ~0.01%). Organism abundance levels were determined based on sequence coverage. Detailed genome reconstructions for the organisms in these samples will be reported separately. Because sequences from the most abundant populations (high sequence coverage) often assemble poorly, the analysis also used two data subsets per sample (1/10th and 1/50th of the data for the GWB1 sample and 1/9th and 1/27th of the data for the GWA1 sample). Community composition analysis used results reconciled from these subassemblies. Genomic data from the subassemblies were binned to specific populations based on GC content, coverage and phylogenetic profile. Each genome was either near-complete or well sampled in one or multiple data sets. Phylogenetic profiling-based binning was helpful because many organisms on the filtrates were relatively similar to organisms that are represented in our in-house candidate phyla genomic data set (WWE3, OP11, OD1 and archaea: reported in refs 14 , 16 , and data to be published elsewhere). Abundances are reported as coverage and/or DNA representation. Coverage was determined based on read mapping statistics. DNA representation used coverage statistics, approximate genome size and total data size (as above). Cryo-TEM specimen preparation in the field For cryo-TEM and synchrotron infrared (SIR) spectromicroscopy (see below), 200 mesh lacey carbon-coated formvar Cu-grids (Ted Pella Inc., Redding, CA, USA) were used. For correlative FISH and TEM, a lacey or a continuous formvar support film was laid on TEM nickel finder grids (Maxtaform Finder Grid Style H7, 63-μm pitch 400 mesh) and grids were carbon coated. All TEM grids were treated by glow discharge to improve sample deposition onto the grids. Ten and 250 nm colloidal gold particles (BBInternational, Cardiff, UK) were put on TEM grids for cryo-TEM and SIR spectroscopy, and for correlative FISH and TEM, respectively, and allowed to dry prior to sample addition. Aliquots of 5 μl 0.2-μm-filtered groundwater sample were deposited onto the grids, manually blotted with filter paper and plunged into liquid propane at liquid nitrogen temperature using a portable cryo-plunge device on site [17] . Grids were stored in liquid nitrogen until further analysis. Clone fluorescence in situ hybridization Subcloning for construction of the positive controls, E. coli cells each carrying the 16S rRNA gene sequence of one of the three bacterial types (WWE3, OP11 and OD1) was performed using the Novagen AccepTor Vector Kit (EMD Millipore, Merck KGaA, Darmstadt, Germany). Subclones with OP11-WWE3-OD1 16S rRNA gene sequences present were identified by sequencing using pETBlueT7UP forward (5′-TCATAACGTCCCGCGAAA-3′) and pETBlueDown reverse (5′-GTTAAATTGCTAACGCAGTCA-3′) primers and BLAST [44] against the Arb-Silva Database. Plasmids containing WWE3-OP11-OD116S rRNA sequences were isolated from subclones used to transform into the NovaBlue (DE3) strain for the subsequent Clone-FISH steps (EMD Millipore, Merck KGaA). Clone-FISH E. coli strains transformed with WWE3-OP11-OD1 sequences were fixed for FISH by centrifuging at 15,000 r.p.m. for 2 min at 4 °C, resuspending in 1 ml PBS (pH 7), centrifuging again and resuspending in 250 μl PBS and 750 μl 4% paraformaldehyde. Cells were allowed to fix for 3 h at 4 °C before centrifuging at 15,000 r.p.m. for 2 min at 4 °C, resuspending in a 1:1 mixture of ethanol and PBS. FISH runs were performed at a range of formamide concentrations between 20 and 50% to establish the optimum concentration that allowed proper hybridization but reduced apparent nonspecific binding. CARD-FISH For correlative cryo-TEM and CARD-FISH two approaches were performed. For the first approach, frozen samples on Ni-Finder TEM grids were imaged and then the CARD-FISH protocol was applied [50] . For the second approach, frozen samples on Ni-Finder TEM grids were freeze-dried and embedded in low-gelling point agarose (0.1% final concentration), dried at room temperature, then fixed in paraformaldehyde solution (2% final concentration), washed in sterile Milli-Q water, dehydrated in 50, 80, 90 and in 100% ethanol and air dried. Three different oligonucleotide probes ( Supplementary Table 8 ), targeting rRNA genes, were applied to cells on TEM grids. Hybridization was performed following a method previously described in ref. 50 , with a formamide concentration of 50%, incubation at 46 °C for 3 h and washing at 48 °C for 10 min. The subsequent amplification was performed at 46 °C for 10 min. Samples were counterstained with 4',6-diamidino-2-phenylindole DNA stain (1 μg ml −1 final concentration). Confocal laser scanning microscopy was performed on a Carl Zeiss Inc. LSM 710 Zen 2010, Release Version 6.0 software (Carl Zeiss MicroImaging Inc., Thornwood, NY, USA), equipped with argon (458 nm, 488 nm and 514 nm) and He–Ne (594 nm, 543 nm and 633 nm) lasers and a diode 45–30 (405 nm). The diode (405 nm) was used for 4',6-diamidino-2-phenylindole signals (BP filter 410–585). Positively labelled cells (fluorochrome Alexa Fluor 546) were detected using the He–Ne 543 nm laser line (BP filter 548–680). A Plan-Apochromat × 100/1.4 oil differential interference contrast (DIC) (Zeiss) lens was used. 2D and 3D cryo-TEM Cryo-TEM images were acquired on a JEOL–3100-FFC electron microscope (JEOL Ltd, Akishima, Tokyo, Japan) equipped with a field emission gun electron source operating at 300 kV, an Omega energy filter (JEOL), cryo-transfer stage and a Gatan 795 4 × 4 K charge-coupled device camera (Gatan Inc., Pleasanton, CA, USA) mounted at the exit of an electron decelerator held at a voltage of 200–250 kV [51] . The stage was cooled with liquid nitrogen to 80 K during acquisition of all data sets. Over 100 2D images were recorded at different magnifications giving a pixel size of 0.375, 0.28 or 0.22 nm at the specimen. Underfocus values ranged between 3.6 μm±0.25 μm and 12 μm±0.5 μm, and energy filter widths were typically around 30 eV. The survey of the grids and the selection of suitable targets were done in low-dose defocused diffraction mode to minimize radiation damage. Thirteen tomographic tilt series were acquired under low-dose conditions, typically over an angular range between +65° and −65°, ±5° with increments of 2°. Between 61 and 66 images were recorded for each tilt series, acquired semi-automatically with the program Serial-EM ( http://bio3d.colorado.edu/ ) [52] adapted to JEOL microscopes. For tilt series data sets, all images show a pixel size of 0.56 or 0.746 nm at the specimen. Underfocus values ranged between 3.6 μm±0.25 μm and 9 μm±0.5 μm, and energy filter widths were ~30 eV. The average dose used per complete tilt series was ~113 e − Å −2 . All tomographic reconstructions were obtained with the program Imod ( http://bio3d.colorado.edu/ ) [52] . The software ImageJ 1.38 × (NIH, http://rsb.info.nih.gov/ij/ ) [53] was used for analysis of the 2D image projections. All movies were created with the open-source package ffmpeg ( http://www.ffmpeg.org/ ). Adobe Photoshop CS5.1 was used to adjust contrast in the images and to insert calibrated scale bars into images. SIR spectromicroscopy Cryo-TEM grids were placed onto the BaF 2 infrared windows (International Crystal Laboratories, NJ, USA) under liquid nitrogen. They were then allowed to air dry at ambient temperature on the BaF 2 windows. SIR spectromicroscopy was performed at the infrared beamline 1.4.3 (Advanced Light Source, http://infrared.als.lbl.gov/ ) on a Nic-Plan infrared microscope ( × 32 objective, numerical aperture=0.65; released software OMNIC 7.0) equipped with a Nicolet Magna 760 infrared spectrometer (Thermo Scientific Inc., MA, USA) at the mid-infrared frequency range (2.5–15.5 μm wavelength, or 4,000–650 cm –1 wavenumber). The infrared signals (in absorbance) from the energy exchange between the infrared photons and biomolecules were sampled by dividing the TEM grid in 2-μm pixels, raster scanned and processed following a method previously described elsewhere [22] , [54] . Cells were detected using the absorption bands of protein amide I and of lipids methyl (−CH 3 ) and methylene (−CH 2 −) groups. Analysis made use of a database of known bacterial and archaeal standards. Accession codes: 16S rRNA gene and ribosomal protein sequences (after acetate amendment) used in the phylogenetic analyses are deposited in the GenBank database under accession codes KC990412 – KC990435 and KC999117 – KC999376 , respectively. How to cite this article: Luef, B. et al. Diverse uncultivated ultra-small bacterial cells in groundwater. Nat. Commun. 6:6372 doi: 10.1038/ncomms7372 (2015).